RETRACTED ARTICLE: Colloidal silver diphosphide (AgP2) nanocrystals as low overpotential catalysts for CO2reduction to tunable syngas Production of syngas with tunable CO/H 2 ratio from renewable resources is an ideal way to provide a carbon-neutral feedstock for liquid fuel production. Ag is a benchmark electrocatalysts for CO 2 -to-CO conversion but high overpotential limits the efficiency. We synthesize AgP 2 nanocrystals (NCs) with a greater than 3-fold reduction in overpotential for electrochemical CO 2 -to-CO reduction compared to Ag and greatly enhanced stability. Density functional theory calculations reveal a significant energy barrier decrease in the formate intermediate formation step. In situ X-ray absorption spectroscopy (XAS) shows that a maximum Faradaic efficiency is achieved at an average silver valence state of +1.08 in AgP 2 NCs. A photocathode consisting of a n + p-Si wafer coated with ultrathin Al 2 O 3 and AgP 2 NCs achieves an onset potential of 0.2 V vs. RHE for CO production and a partial photocurrent density for CO at −0.11 V vs. RHE ( j −0.11, CO ) of −3.2 mA cm −2 . Syngas with a tunable CO/H 2 ratio is a particularly attractive commodity because it can subsequently be upgraded to synthetic liquid fuels by industrial Fischer–Tropsch reactions [1] . Currently, non-renewable fossil fuels are the predominant sources for syngas production, all of which contribute to environmental pollution [2] . The conversion of CO 2 into value-added chemicals by use of renewable energy (e.g. solar energy) is an ideal approach to achieving a carbon-neutral energy cycle [3] , and the development of an efficient and selective catalyst is critical to make this technology feasible. For most metallic CO 2 reduction catalysts, both theory and experiment have shown that only an H 2 -rich mixture is achievable because the HER process dominates in aqueous solution [4] . Au and Ag have emerged as benchmark electrocatalysts for highly selective conversion of CO 2 to CO [5] . Compared to the Au electrocatalyst, Ag is considerably cheaper and shows comparable activity. Various strategies, such as morphology-nanostructuring [6] , [7] , size-tuning [8] , defect-engineering [9] , surface ligand functionalization [10] , and bimetal alloying [11] , have been utilized to decrease the required overpotential ( η ) for high selectivity of CO 2 -to-CO on Ag-based electrocatalysts. However, Ag still suffers from a high overpotential and the current density of syngas at low overpotential ( η < 500 mV) is usually below a metric value of 10 mA/cm 2 . Moreover, the ratio of CO:H 2 is generally limited to the range of 1:2 to 1:1, severely restricting the flexibility for integration with existing chemical infrastructure. Incorporation of non-metal elements such as phosphorus, sulfur, and boron into metals to form multicomponent alloys is an effective way to tailor the electronic structure and surface properties of metal electrocatalysts [12] , [13] , [14] . Our previous work studying the hydrogen evolution reaction (HER) on CoP found that phosphorus was able to regulate the binding strength of reaction intermediates adsorbed on cobalt active sites to improve electrocatalytic activity [15] . While silver diphosphide (AgP 2 ) is an attractive material for electrocatalysis given the success of other metal phosphide systems, it is rarely reported due to a lack of synthetic methods to control the nanostructured morphology and purity [16] , [17] . Colloidal synthesis has been shown to yield high monodispersity with controllable morphology but only limited work has been done on noble metal phosphide (e.g. AgP 2 ) NCs and they have not been employed for CO 2 reduction [18] . It is highly desirable to understand how the incorporation of P into Ag affects the catalytic efficiency, stability, and selectivity for CO 2 reduction applications. One attractive method for converting solar energy into chemical fuels is via photoelectrochemical (PEC) conversion. However, overall PEC device performance still suffers from the limitations of high overpotential, poor selectivity, and instability in the long-term operation [19] . Rational design is required to optimize the interface between semiconductor and cocatalyst for efficient charge transfer, and a catalyst that exhibits a fast reaction rate at low overpotential while maintaining high selectivity. Recently, a wide range of semiconductors, such as p-Si [20] , [21] , CuFeO 2 /CuO [22] , ZnTe [23] , [24] , and GaN [25] have been studied in PEC CO 2 reduction to produce CO or formate. These semiconductors are typically paired with an effective and selective metal cocatalyst such as Au, Ag, and Cu. For efficient PEC CO 2 reduction, selective cocatalysts are generally integrated with a p-type semiconductor. P-type silicon (p-Si) is one of the most promising candidates for PEC CO 2 reduction due to its narrow band gap (1.1 eV) and abundance [26] . Incorporation of a high level of surface n-dopant can decouple the band bending in the p-Si from the semiconductor-liquid junction to form an n + p built-in depletion region, which increases the photovoltage of the p-Si photocathode [27] . However, direct contact between n + p-Si and a metal cocatalyst can lead to severe surface recombination due to Fermi level pinning, lowering the built-in photovoltage [28] . Inserting an ultrathin insulator layer to form a buried heterojunction can eliminate Fermi level pinning and provide a higher photovoltage to drive the chemical reaction, while also protecting the semiconductor from the corrosive electrolyte. Ultrathin and pin-hole free metal oxides have been fabricated by atomic layer deposition (ALD) and used as tunnel layers for efficiently mediating charge transfer from semiconductor to cocatalyst [29] , [30] , [31] . In the past few years, photoelectrodes with buried junction have been investigated in PEC water splitting [32] , [33] , [34] , [35] but have not been realized in PEC CO 2 reduction for syngas production due to the lack of efficient and selective metal cocatalysts. Synthesis and characterization of AgP 2 nanocrystals To synthesize monodisperse and crystalline silver phosphide NCs, a reactive phosphorus precursor is key for achieving the necessary balance of Ag + reduction and P incorporation. The use of trioctylphosphine (TOP) requires a high temperature (>280 °C) to achieve TOP decomposition to generate the PH 3 intermediate [36] . For silver phosphide NCs synthesis, the reduction rate for Ag + to Ag is too fast at high temperature and severe aggregation and precipitation occurs [37] . Tris(trimethylsilyl)phosphine (P(SiMe 3 ) 3 ) is an alternative to in situ PH 3 generation, opening a wider temperature window. 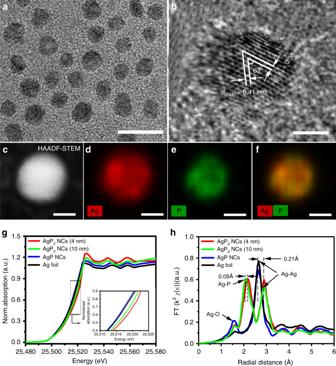Fig. 1 Materials characterization of AgP2NCs.aTEM image, scale bar 10 nm.bHRTEM image,cHAADF-STEM,d–felemental mapping images of AgP2NCs. Scale bars 2 nm.gX-ray absorption near-edge structure (XANES) spectra of 4 nm AgP2NCs, 10 nm AgP2NCs, 10 nm Ag NCs, and Ag foil.hCorresponding extended X-ray absorption fine structure (EXAFS) spectra. High-quality silver phosphide NCs are obtained by hot-injection at 180 °C, maintaining the temperature for 10 min, then fast cooling to 80 °C where the temperature is held for 60 min Inductively coupled plasma mass spectroscopy (ICP-MS) gives an atomic ratio of silver to phosphorus of 0.505, consistent with AgP 2 (Supplementary Table 1 ). Energy-disperse X-ray spectroscopy (EDS) of AgP 2 shows a similar Ag:P ratio of 0.517 (Supplementary Fig. 1 ). The X-ray diffraction (XRD) pattern of AgP 2 NCs is highly matched with the monoclinic structure (ICDD PDF: 01-018-1185) (Supplementary Fig. 2 ), and notably does not show the existence of a crystalline Ag impurity in the silver phosphide NCs. The central Ag atom is octahedrally coordinated by P atoms, while P atoms are tetrahedrally coordinated by P and Ag atoms (Supplementary Fig. 3 ). The P-rich composition distorts the Ag cubic structure and potentially leads to exposure of abundant uncoordinated sites to be exploited for catalysis. The transmission electron microscopy (TEM) image of the as-synthesized AgP 2 NCs shows a relatively uniform spherical morphology with the average size of 3.5 ± 0.5 nm (Fig. 1a ). Two sets of lattice fringes are observed, showing interplane distances of 0.41 and 0.39 nm corresponding to the (011) and ( \(\bar 1\) 02) planes of the monoclinic AgP 2 (Fig. 1b ). The intersected angle between the (011) and ( \(\bar 1\) 02) planes is 63°, very close to the monoclinic theoretical value of 65°. The two lattice fringes are also found in the selected-area electron diffraction (SAED) image and fast Fourier transform (FFT) image (Supplementary Fig. 4 ). To better understand the effects of ultrasmall NC size, AgP 2 NCs with a larger size of around 10 nm were obtained by extending the reaction time at 180 °C to 25 min. For the 10 nm AgP 2 NCs, only a general (111) plane is presented on nanocrystal surface (Supplementary Fig. 5a, b ), indicating the critical role of controlling nanocrystal size on enhancing the exposure of high-index planes which may exhibit higher catalytic activity [8] . High-angle annular dark-field scanning TEM (HAADF-STEM) image shows a single AgP 2 NC that possesses well-defined spherical geometry (Fig. 1c ). Figure 1d–f show the elemental mapping of an individual AgP 2 NC obtained by HAADF-STEM-EDS, in which the Ag and P elements are evenly distributed throughout the whole NC. Fig. 1 Materials characterization of AgP 2 NCs. a TEM image, scale bar 10 nm. b HRTEM image, c HAADF-STEM, d – f elemental mapping images of AgP 2 NCs. Scale bars 2 nm. g X-ray absorption near-edge structure (XANES) spectra of 4 nm AgP 2 NCs, 10 nm AgP 2 NCs, 10 nm Ag NCs, and Ag foil. h Corresponding extended X-ray absorption fine structure (EXAFS) spectra. Full size image X-ray absorption spectroscopy further reveals the effect of phosphorus incorporation on the local geometric and electronic structures of silver in AgP 2 NCs. Figure 1g shows the Ag K-edge X-ray absorption near-edge structure (XANES) spectra of 4 nm AgP 2 NCs, 10 nm AgP 2 NCs, 10 nm Ag NCs, and Ag foil. The rising edge of AgP 2 NCs shows a positive shift compared with that of Ag NCs due to the increased Ag valence oxidation state after incorporation of P into Ag. This can be ascribed to an electron density shift from Ag to P-rich regions with high electronegativity [38] . The X-ray photoelectron spectroscopy (XPS) binding energy (Supplementary Fig. 6 ) of Ag 3 d 5/2 for AgP 2 NCs is positively shifted (0.7 eV) from that of Ag 3 d 5/2 for Ag NCs, while there is negative shift for the binding energy of P 2 p 3/2 (128.6 eV) in AgP 2 NCs when compared to that of elemental P (130.0 eV) [15] . The white line intensity for AgP 2 NCs is stronger than that for Ag NCs, which indicates a decrease in the number of electrons in the Ag frontier orbitals [39] . Moreover, decreasing the size of AgP 2 NCs leads to increases of both rising edge intensity and white line intensity, which are ascribed to the changes of coordination environment and surface states [40] . The Fourier transforms of the k 3 -weighted extended Ag K-edge X-ray absorption fine structure (EXAFS) spectra were shown in Fig. 1h . The EXAFS fitting results are summarized in Supplementary Fig. 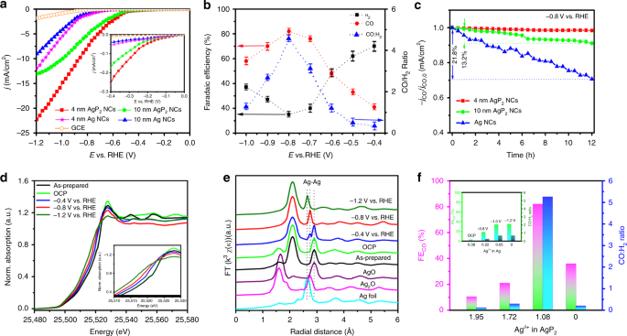Fig. 2 Electrochemical measurements in CO2-saturated 0.5 M KHCO3solution.aLinear sweep voltammetric curves;bFaradaic efficiency of CO and H2and CO/H2ratio;cstability of partial CO current density (jCO) measured at −0.8 V vs. RHE for 12 h.dIn situ silver K-edge XANES andeEXAFS spectra of 4 nm AgP2NCs after 30 min at the specified potential. Pristine AgP2NCs, AgO, Ag2O, and Ag foil are included as references.fFaradaic efficiency of the CO and CO:H2ratio as a function of Agδ+in AgP2and Ag. 7 and Table 2 . The Ag–Ag bond length for AgP 2 NCs is larger than that for Ag NCs and Ag foil (2.65 Å), which is ascribed to the negatively charged P-rich clusters strongly binding the surrounding Ag atoms and thus weakening the Ag–Ag bonding strength. The P incorporation into Ag also results in a decrease of coordination numbers of Ag–Ag and structural disorder (Supplementary Table 2 ). Electrochemical CO 2 reduction The CO 2 electroreduction performance of 4 nm AgP 2 NCs was measured in a Nafion membrane-separated H-type cell. For comparison, the performance of 10 nm AgP 2 NCs, 4 nm Ag NCs, and 10 nm Ag NCs were also measured. The gaseous and liquid products were determined by a gas chromatography (GC) and H 1 NMR, respectively, and only CO and H 2 were observed. 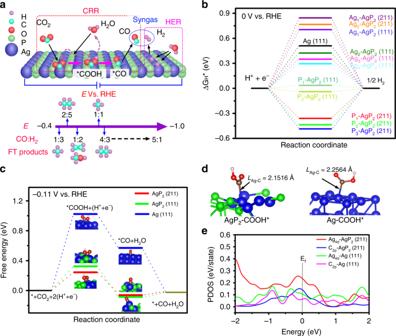Fig. 3 Density functional theory calculations.aSchematic diagram of selective CO2-to-syngas on AgP2(211). Free energy change (ΔG) calculated for thebHER andcselective CO2-to-CO reaction.dOptimized *COOH adsorption configuration andecorresponding PDOS on AgP2(211) and Ag (111). The geometric current density, CO and H 2 Faradaic efficiency, and CO partial current density as a function of potential for 4 nm AgP 2 NCs are summarized in Supplementary Table 3 . Figure 2a shows the polarization curves acquired in a CO 2 -saturated 0.5 M KHCO 3 . The 4 nm AgP 2 NCs achieve a current density as high as −15.2 mA cm −2 at −1.0 V vs. RHE, over twice that of 4 nm Ag NCs, and 3.6 times higher than that of 10 nm Ag NCs. The enhanced overall electrochemical activity of the 4 nm AgP 2 NCs is potentially related to increased electrochemical active surface area (EASA) and interfacial charge transfer rate (Supplementary Figs. 8a and 9 ). The onset potential ( E onset, CO ) for initial CO generation (defined as the potential required for j CO = −0.01 mA cm −2 ) on 4 nm AgP 2 NCs is −0.22 V vs. RHE, which is only 110 mV lower than the thermodynamic potential of CO 2 -to-CO reaction. In comparison, the E onset, CO for Ag NCs is −0.59 V vs. RHE ( η = 480 mV). The 4 nm AgP 2 NCs exhibit an overpotential for the same partial density of CO ( j CO ) that is consistently on the order of 0.3 V lower than 10 nm Ag NCs (Supplementary Fig. 10 ). The source of the anodic shift of onset potential and decreased overpotential for CO 2 -to-CO will be discussed below in detail. The performance of 10 nm AgP 2 NCs is also provided as a same-size comparison to 10 nm Ag NCs, and also exhibit uniformly superior performance compared to Ag NCs. 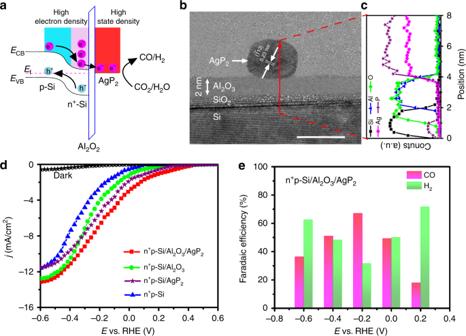Fig. 4 Photoelectrochemical device and performance.aSchematic energy level alignment.bCross-sectional HRTEM image of n+p-Si/Al2O3/AgP2hybrid photocathode andccorresponding line scan elemental EDS spectra. Scale bar 5 nm.dj–Ecurves of as-prepared n+p-Si, n+p-Si/AgP2, n+p-Si/Al2O3, and n+p-Si/Al2O3/AgP2photocathodes under simulated solar illumination (AM-1.5G, 100 mW cm−2) in CO2-saturated 0.5 M KHCO3solution.eFaradaic efficiency of CO and H2at different potentials for n+p-Si/Al2O3/AgP2. Notably, the 4 nm AgP 2 NCs exhibit a remarkable geometric j CO of −0.27 and −8.7 mA cm −2 at −0.5 and −1.0 V vs. RHE, respectively, which is the one of the highest values reported for Ag-based electrocatalysts for CO 2 reduction (Supplementary Table 4 ). A maximum FE CO of 82% and minimum FE H2 of 15% is simultaneously achieved at −0.8 V vs. RHE (Fig. 2b ), indicating CO 2 -to-CO reduction is more favorable than the competitive HER on 4 nm AgP 2 NCs. The CO:H 2 ratio in the syngas product varies from 1:3 to 5:1 in the potential range of −0.4 to −1.0 V vs. RHE. This is the widest range of syngas proportions for all Ag-based electrocatalysts (Supplementary Table 4 ), and even superior or comparable to recently reported electrocatalysts with impressive syngas efficiency, such as Au–Cu (1:2 to 4:1) [41] , Pd/C (1:4 to 1:1) [42] , Co 3 O 4 -CDots-C 3 N 4 (1:4 to 14:1) [43] , MoSeS (1:3 to 1:1) [44] , and CdS x Se 1− x (1:4 to 4:1) [45] . Notably, the 4 nm AgP 2 NCs achieve all the key syngas ratios with nearly 100% Faradaic efficiency within an overpotential of 500 mV at stability for 12 h (Supplementary Table 3 , Supplementary Fig. 11 ). The contribution to the H 2 from catalyst substrates (Ketjet carbon or glassy carbon) was characterized and is minimal below −0.8 V vs. RHE (Supplementary Fig. 12 ). For comparison, a much lower FE CO,max and narrower CO:H 2 range is observed for Ag NCs (Supplementary Tables 6 and 7 ). To check that the NC surface is exposed, the effects of removing surface capping ligands on the electrochemical surface area and FE CO are shown in Supplementary Fig. 13a–c . The Tafel slope for 4 nm AgP 2 NCs, 10 nm AgP 2 NCs, 4 nm Ag NCs, and 10 nm Ag NCs is 105, 117, 168, and 184 mV/dec, respectively (Supplementary Fig. 14 ). The smallest Tafel slope for 4 nm AgP 2 NCs indicates that phosphorus plays a critical role in stabilizing the CO 2 - intermediate and accelerating the first electron transfer rate-determining step [6] . Additionally, the durability of 4 nm AgP 2 NCs, 10 nm AgP 2 NCs, and 10 nm Ag NCs was tested at a high constant potential of −0.8 V vs. RHE (Fig. 2c ). A stable j CO with negligible decay within 12 h is observed on 4 nm AgP 2 NCs, compared to 13.2% and 21.8% activity decay for 10 nm AgP 2 NCs and Ag NCs, respectively. ICP-MS, TEM, and XPS confirm that the 4 nm AgP 2 NCs remain almost the same after 12 h CO 2 reduction (Supplementary Figs. 15 – 17 ). Fig. 2 Electrochemical measurements in CO 2 -saturated 0.5 M KHCO 3 solution. a Linear sweep voltammetric curves; b Faradaic efficiency of CO and H 2 and CO/H 2 ratio; c stability of partial CO current density ( j CO ) measured at −0.8 V vs. RHE for 12 h. d In situ silver K-edge XANES and e EXAFS spectra of 4 nm AgP 2 NCs after 30 min at the specified potential. Pristine AgP 2 NCs, AgO, Ag 2 O, and Ag foil are included as references. f Faradaic efficiency of the CO and CO:H 2 ratio as a function of Ag δ+ in AgP 2 and Ag. Full size image To gain insight into the electronic structure and relationship between the chemical state of the 4 nm AgP 2 NCs and the catalytic selectivity during CO 2 electroreduction, operando XANES and EXAFS measurements were carried out under various applied potentials for 30 min in aqueous CO 2 -saturated 0.1 M KHCO 3 (Fig. 2d, e ). Commercial AgO, Ag 2 O, and Ag foil were used as references and a linear combination of XANES spectra was fitted to the in situ Ag K-edge spectra (Supplementary Fig. 18 ). The absorption edge (E 0 ) and corresponding oxidation state of the silver species in AgP 2 under various potentials are summarized in Supplementary Table 8 . For the as-prepared AgP 2 NCs, the absorption edge and radial distance of Ag–Ag are close to that of the AgO sample, and the initial oxidation state of the silver species is calculated to be +1.96. Under open-circuit potential (OCP), the oxidation state remains the same. When the applied potential increases to −0.4 V vs. RHE, the absorption edge shows a negative shift and a small Ag–Ag peak appears at the radial distance of 2.74 Å, suggesting the AgP 2 is partially reduced and the average oxidation state decreases to +1.72. At the potential of −0.8 V vs. RHE, which corresponds to the peak in selectivity for CO 2 -to-CO, the oxidation state of the silver species is further reduced to +1.08. The evolution of the silver oxidation state in AgP 2 from +1.96 to +1.08 occurs rapidly within 2 min under applied potential of −0.8 V vs. RHE and remains stable for 2 h. In comparison, AgO and Ag 2 O are reduced to Ag 0 in less than 50 s at −0.8 V vs. RHE (Supplementary Fig. 19 ), which suggests that the rich-P content is beneficial to stabilize Ag +1.08 . Maintaining this positive oxidation state under a highly reductive potential may be the key to the lowered the activation barrier of the initial CO 2 reduction step and the stable and selective production of CO 2 -to-CO at −0.8 V. If the applied potential goes further to −1.2 V vs. RHE, the spectrum is matched with the Ag foil, indicating a complete transition from Ag +1.08 to Ag 0 . The operando measurements suggest phosphorus can stabilize a relatively high silver oxidation state which is critical to high FE CO and wide CO:H 2 range within a low overpotential window (Fig. 2f ). Theoretical investigation of intermediates The schematic diagram of CRR and HER processes for tunable syngas production is summarized in Fig. 3a , where the ratio of syngas can be tuned over a wide range by changing applied potentials to meet input ratios necessary for the Fischer-Tropsch synthesis of hydrocarbons and alcohols. Silver-based CO 2 reduction electrocatalysts generally follow two hydrogenation steps plus one nonelectrochemical CO desorption, i.e., \({\mathrm{CO}}_2 \to \ast {\mathrm{COOH}} \to \ast {\mathrm{CO}} \to {\mathrm{CO}}\) . Density functional theory (DFT) was used to understand the key role of phosphorus alloying on the low overpotential and highly tunable syngas ratio observed on AgP 2 NCs relative to Ag NCs. Low index (111) and high-index (211) facets were selected as representative surfaces for AgP 2 [46] . Since HER is a competitive process with CO 2 reduction reaction (CRR) in aqueous solution, DFT calculation was initially used to determine the free energy for atomic hydrogen adsorption (Δ G H* ) on AgP 2 and Ag electrocatalysts. The calculated ΔG H* on AgP 2 (211), AgP 2 (111), and Ag (111) surfaces are shown in Fig. 3b and corresponding complete structures and energies are provided in Supplementary Fig. 21 and Table 9 . The closed packed Ag (111) surface exhibits a large positive ΔG H* of 0.510 eV, which implies a high-energy barrier for hydrogen adsorption process, consistent with previously reported Ag-based HER catalysts [47] . For AgP 2 (211) and AgP 2 (111), weak absorption of atomic H* on silver is still observed, with an average Δ G H* of 0.806 and 0.443 eV for AgP 2 (211) and AgP 2 (111), respectively. However, the HER process can proceed via P sites, and the AgP 2 (111) surface has P sites (denoted P 1 and P 2 ) with a Δ G H* of 0.036 and −0.039 eV, favorable for hydrogen production. Interestingly, for the high-index surface AgP 2 (211), all three P HER active sites (denoted as P 1 , P 2 , and P 3 ) have much lower Δ G H* values (−0.360, −0.436, and −0.486 eV, respectively). Not only will strong adsorption of H* on phosphorus sites suppress the HER rate, but the adsorbed H* may also be delivered to the adsorbed carbon species on adjunct silver sites to promote the hydrogenation reaction. Fig. 3 Density functional theory calculations. a Schematic diagram of selective CO 2 -to-syngas on AgP 2 (211). Free energy change (Δ G ) calculated for the b HER and c selective CO 2 -to-CO reaction. d Optimized *COOH adsorption configuration and e corresponding PDOS on AgP 2 (211) and Ag (111). Full size image The optimized geometrics of *COOH and *CO intermediates on AgP 2 (211), AgP 2 (111), and Ag (111) surfaces and corresponding adsorption energy are included in Supplementary Fig. 22 and Table 10 . Figure 3b depicts the free energy diagram for the lowest free energy path for the selective CO 2 -to-CO pathway at an equilibrium potential of −0.11 V vs. RHE. For all three surfaces, the initial CO 2 hydrogenation is the rate-determined step for the CO 2 -to-CO process; however Δ G *COOH for both AgP 2 surfaces is over threefold lower than that for Ag. This is in excellent agreement with the experimentally observed decrease in the overpotential for CO 2 reduction. The minimal applied potential ( U mp ) for CO 2 -to-CO reduction on AgP 2 (211), AgP 2 (111), and Ag (111) is determined as −0.355, −0.434, and −1.134 V vs. RHE, respectively (Supplementary Fig. 23 ). This theoretical U mp is of greater magnitude than the experimental E onset,CO on 4 nm AgP 2 NCs of −0.22 V vs. RHE, indicating non-thermodynamic factors might be involved in lowering the activation energy barrier of the first hydrogenation process. At the same time, CO remains only weakly adsorbed on AgP 2 with a binding free energy of around 0.085 eV. While CO is bound more tightly for AgP 2 than for Ag, it is far from the strong adsorption regime that causes catalyst poisoning for Pt-based catalysts where binding strength on the order of −1 eV [48] . Comparing the 4 nm AgP 2 NCs versus 10 nm AgP 2 NCs, the higher electrocatalytic performance and ability to achieve high CO content syngas for the 4 nm AgP 2 is consistent with the enhanced presence of high-index planes such as (211) on the ultrasmall NCs [8] . Analysis of the partial density of states (PDOS) and Bader charge is used to understand the role of P in increasing the binding to Ag. PDOS shows that in AgP 2 the valence Ag 4 d orbital is more delocalized with higher density d -valence band states compared to Ag at the Fermi level (Fig. 3e ). This leads to a higher overlap between Ag 4 d and C 2 p , consistent with stronger *COOH adsorption [49] . The Ag–C bond lengths of 2.15 Å for AgP 2 is shorter than that for Ag (Fig. 3d ), suggesting tighter binding of *COOH on AgP 2 . Bader charge analysis shows that the bond strength increases with the partial positive charge on Ag, with the most stable *COOH adsorption site on AgP 2 (211) having a Bader charge of Ag 0.2+ compared to metallic Ag 0 sites [50] . Hybrid photocathode for PEC Inspired by the efficient activity, selectivity, and stability of 4 nm AgP 2 NCs toward syngas from CO 2 electroreduction, we integrated 4 nm AgP 2 NCs onto a surface-protected n + p-Si semiconductor to build a hybrid photocathode of n + p-Si/Al 2 O 3 /AgP 2 based on the buried junction design. Briefly, an ultrathin 2 nm Al 2 O 3 layer was deposited by ALD to protect the underlying silicon semiconductor from electrolyte corrosion and eliminate the potential for additional interfacial resistance due to in situ growth of silicon oxide. Diluted 4 nm AgP 2 NCs were deposited using spin coating without any aggregation (Supplementary Fig. 24 ). The mechanism for PEC CO 2 reduction is depicted in Fig. 4a and begins with the photogenerated minor carrier electrons in n + p-Si accumulating at the n + p-Si/Al 2 O 3 interface. The Al 2 O 3 is kept thin enough to allow efficient electron tunneling into the AgP 2 cocatalyst, and selective CO 2 electroreduction occurs at the AgP 2 surface. The work function of AgP 2 NCs (4.2 eV) is smaller than that of Ag NCs (4.8 eV) and AgP 2 NCs are metallic. (Supplementary Fig. 25 and Fig. 26 ). Figure 4b shows a cross-sectional high-resolution transmission electron microscopy (HRTEM) image of the n + p-Si/Al 2 O 3 /AgP 2 interface. The corresponding elemental distribution from STEM-EDS line scan across the n + p-Si/Al 2 O 3 /AgP 2 interface is shown in Fig. 4c . The Al signal is evident at the interface between the Si and Ag signal. The Si semiconductor and AgP 2 cocatalyst are well separated by the Al 2 O 3 layer, which is expected to help passivate and protect the Si surface [28] . The n + p-Si/Al 2 O 3 /AgP 2 shows similar absorption (Supplementary Fig. 27 ) compared with n + p-Si and n + p-Si/Al 2 O 3 , indicating the negligible light absorption and reflection loss from the ultrathin ALD oxide and sparse AgP 2 nanocrystal layer. Fig. 4 Photoelectrochemical device and performance. a Schematic energy level alignment. b Cross-sectional HRTEM image of n + p-Si/Al 2 O 3 /AgP 2 hybrid photocathode and c corresponding line scan elemental EDS spectra. Scale bar 5 nm. d j – E curves of as-prepared n + p-Si, n + p-Si/AgP 2 , n + p-Si/Al 2 O 3 , and n + p-Si/Al 2 O 3 /AgP 2 photocathodes under simulated solar illumination (AM-1.5G, 100 mW cm −2 ) in CO 2 -saturated 0.5 M KHCO 3 solution. e Faradaic efficiency of CO and H 2 at different potentials for n + p-Si/Al 2 O 3 /AgP 2 . Full size image Figure 4d shows the current density vs. potential ( j – E ) curves of the as-prepared n + p-Si/Al 2 O 3 /AgP 2 photocathode in a CO 2 -saturated 0.5 M KHCO 3 solution under simulated AM-1.5G solar illumination. Under dark condition, the n + p-Si/Al 2 O 3 /AgP 2 shows a very negative onset potential of −0.16 V vs. RHE (defined as the potential to attain a total current of −0.1 mA cm −2 ) and negligible current in the potential window. Under illumination, n + p-Si/Al 2 O 3 /AgP 2 exhibits the most positive onset potential ( E onset = 0.42 V vs. RHE) compared to control devices in which select layers are missing: n + p-Si/Al 2 O 3 (0.28 V vs. RHE), n + p-Si/AgP 2 (0.31 V vs. RHE), and n + p-Si (0.12 V. RHE). The photovoltage for n + p-Si/Al 2 O 3 /AgP 2 is around 580 mV, as estimated by the difference in potential required to achieve −0.1 mA cm −2 under dark versus illumination. This high output photovoltage is superior or comparable to state-of-the-art p-Si photocathodes, such as Ni-Mo/n + p-Si NW (560 mV) [51] , CoP-n + p Si (580 mV) [52] , and p-Si/NiCoSe x [53] (500 mV). The high photovoltage is attributed to (1) the ultrathin Al 2 O 3 overlayer passivating the surface states of n + p-Si and increasing the output photovoltage [34] , and (2) the AgP 2 acting as a cocatalyst for lowering the reaction barrier and providing a fast interfacial reaction rate. However, the saturated photocurrent density ( j sat ) of n + p-Si/Al 2 O 3 /AgP 2 is lower than that (~−30 mA cm −2 ) of an ideal state-of-the-art Si-based photocathode, which is ascribed to the non-ideal p–n homojunction and the Si/Al 2 O 3 interface (Supplementary Fig. 28 ). At the CO 2 -to-CO reduction potential of −0.11 V vs. RHE, n + p-Si/Al 2 O 3 /AgP 2 achieves a total current density ( j −0.11, total ) of −5.2 mA cm −2 . The remarkable j −0.11, total is higher than that of the other photocathodes towards CO 2 reduction, such as Au 3 Cu NP/Si NW ( j −0.11,total = −2.2 mA cm −2 ) [20] , RA-Au/n + p-Si ( j −0.11,total = −4.0 mA cm −2 ) [21] , N:C/N:ZnTe ( j −0.11,total = −1.2 mA cm −2 ) [54] , and Cu-ZnO/GaN/n + p-Si ( j −0.11,total = −1.2 mA cm −2 ) [55] . The Faradaic efficiency for H 2 and CO in the potential range from −0.6 to 0.2 V vs. RHE is summarized in Fig. 4e and Supplementary Table 11 . Detectable CO (FE CO = 18%) starts to be observed at 0.2 V vs. RHE ( E onset, CO ) for n + p-Si/Al 2 O 3 /AgP 2 , while the E onset, CO negatively shifts to 0.09 V vs. RHE for n + p-Si/Al 2 O 3 /Ag, indicating that AgP 2 is more suitable as a cocatalyst for CO 2 -to-CO than Ag, consistent with the CRR results presented above. The n + p-Si/Al 2 O 3 /AgP 2 simultaneously shows a maximum FE CO of 67% and minimum FE H2 of 31% at −0.2 V vs. RHE. When further increasing the applied potential, the FE CO is decreased due to the limitation of CO 2 mass transport and hydrogen evolution becomes the dominant reaction. In the potential window from −0.6 to 0.2 V vs. RHE, the CO/H 2 ratio in the PEC syngas product can be tuned in a large range of 1:5 to 2:1. For the hybrid n + p-Si/Al 2 O 3 /AgP 2 photocathode, it is challenging to determine the fraction of H 2 generated from the AgP 2 catalytic sites rather than the bare n + p-Si/Al 2 O 3 photoelectrode; however, comparing the activity of different surfaces suggests the majority of H 2 is from AgP 2 NCs (Supplementary Figs. 29 and 30 , Table 13 ). Notably, the impressive E onset, CO and partial photocurrent density for CO at −0.11 V vs. RHE ( j −0.11, CO = −3.2 mA cm −2 ) are the best values among all the reported photocathodes for CO 2 reduction (detailed comparison is in Supplementary Table 14 ). The stability for PEC CO 2 reduction was tested at a constant potential of −0.2 V vs. RHE for 12 h (Supplementary Fig. 31 ). Only a minimal change is observed in both total photocurrent density and FE CO during long-term measurement. The incident photon-to-current conversion efficiency (IPCE) of n + p-Si/Al 2 O 3 /AgP 2 reaches a maximum of 67% at 680 nm, while the absorbed photon-to-current conversion efficiency, calculated using the absorption, reflection, and transmission data from Supplementary Fig. 27 , reaches a maximum of 85% (Supplementary Fig. 32 ). The addition of 1-butyl-3-methylimidazolium (BMIM-BF 4 ) ionic liquid into the 0.5 M KHCO 3 solution, an enhanced FE CO of 89% at −0.2 V vs. RHE is reached (Supplementary Table 14 ). The adsorbed BMIM-BF 4 on the catalysts surface lowers the energy barrier for reducing CO 2 to CO 2 ˙ ˉ , enhancing CO production while simultaneously suppressing hydrogen evolution [56] , [57] . The critical roles of each layer in the buried junction structure are revealed by comparison to structures with a component missing. While n + p-Si/Al 2 O 3 is expected to be active for HER, no CO is detected in gas products for both n + p-Si and n + p-Si/Al 2 O 3 within the overpotential of 400 mV because hydrogen evolution is more favorable than CO 2 reduction without the selective cocatalyst (Supplementary Table 12 ). For the n + p-Si/AgP 2 photocathode without the protective ALD layer, a more negative E onset,CO is observed compared to n + p-Si/Al 2 O 3 /AgP 2 (Supplementary Table 14 ), confirming the role of Al 2 O 3 in ensuring high photovoltage output. Further, a 75% photocurrent decay is observed during the stability test of n + p-Si/AgP 2 (Supplementary Fig. 31 ), which is attributed to either etching or an in situ increase in the thickness of the silicon oxide insulator. Interfacial charge transport Cyclic voltammograms (CVs) in ferri/ferrocyanide redox solution elucidate charge transfer in the as-prepared photocathodes as shown in Fig. 5a . Under dark conditions, only an oxidation peak is present in the CV curve of n + p-Si/Al 2 O 3 /AgP 2 . The lack of a reduction peak can be explained by the absence of electrons at the solid electrode/electrolyte interface for Fe (III) reduction or water reduction [32] , [58] . In contrast, a symmetric CV curve with narrow peak-to-peak splitting (61 mV) and a positive shift (380 mV) in the anodic oxidation peak is observed under illumination, indicating the photogenerated electrons are driven to the solid/electrolyte interface and participate in Fe(III) reduction. Without AgP 2 , n + p-Si/Al 2 O 3 exhibits less peak current and wider peak-to-peak splitting (590 mV), suggesting the role of AgP 2 in accelerating the interfacial reaction rate. Increasing the thickness of Al 2 O 3 beyond the 2 nm optimal thickness results in a decrease in the reduction and oxidation peaks due to reduced tunneling through the passivation layer (Supplementary Table 15 ) [28] . For 0.5- and 1-nm- thick Al 2 O 3 layers there is a large reduction in peak current after 10 CV cycles due to incomplete protection of the n + p-Si (Supplementary Fig. 35 ). Fig. 5 Detailed characterization of photoelectrochemical response. a Cyclic voltammogram of n + p-Si/2 nm Al 2 O 3 , n + p-Si/2 nm Al 2 O 3 /AgP 2 , and n + p-Si/5 nm Al 2 O 3 /AgP 2 in ferri/ferrocyanide redox solution. All measurements were conducted in the simulated light illumination except as marked. b In situ transient absorption spectra of as-prepared samples measured in CO 2 -saturated 0.5 M KHCO 3 solution under open-circuit potential. The samples were excited by 450 nm laser with a power of 50 µW. Full size image In situ transient absorption (TA) spectroscopy is a useful tool to understand interfacial charge transfer processes for PEC water oxidation and reduction [59] . However, there are few TA studies of photocathodes for PEC CO 2 reduction due to the timescale mismatch between charge transfer and the surface catalysis process [60] . 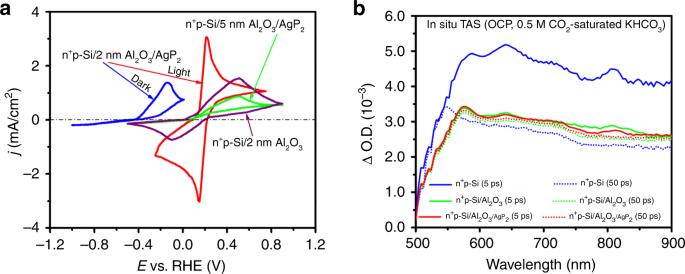Fig. 5 Detailed characterization of photoelectrochemical response.aCyclic voltammogram of n+p-Si/2 nm Al2O3, n+p-Si/2 nm Al2O3/AgP2, and n+p-Si/5 nm Al2O3/AgP2in ferri/ferrocyanide redox solution. All measurements were conducted in the simulated light illumination except as marked.bIn situ transient absorption spectra of as-prepared samples measured in CO2-saturated 0.5 M KHCO3solution under open-circuit potential. The samples were excited by 450 nm laser with a power of 50 µW. Figure 5b shows the in situ TA spectra of as-prepared photocathodes immersed in CO 2 -saturated 0.5 M KHCO 3 solution at OCP. Most notable is the difference in timescales between the n + p-Si sample and the samples passivated with Al 2 O 3 . For bare n + p-Si, between 5 and 50 ps the photogenerated charge carriers are trapped reducing the absorption signal. The wide absorption peak at 580 nm blueshifts to 550 nm and narrows, which is ascribed to electrons relaxing into deep lying localized states [61] . For the samples coated by ALD, only a slight change in OD is observed between 5 and 50 ps and so slow TA spectra (Supplementary Fig. 36 ) were measured. The normalized decay trace for bare n + p-Si yields a representative lifetime ( t 1/2 ) of 3.5 ps, which is over five orders of magnitude shorter than that of n + p-Si/Al 2 O 3 (3.2 µs) and n + p-Si/Al 2 O 3 /AgP 2 (6.3 µs). In TA absorption spectra (at 1 ms) of n + p-Si and n + p-Si/Al 2 O 3 /AgP 2 at an applied potential of −0.2 V vs. RHE (Supplementary Fig. 37 ), unmodified n + p-Si/Al 2 O 3 exhibits a TA spectrum peaking at 610 nm. After AgP 2 decoration, the amplitude at 610 nm is lost, and a new peak appears at 690 nm, which suggests efficient electron transfer from the n + p-Si/Al 2 O 3 surface to AgP 2 [62] . Transient photocurrent (TPC) measurements were carried out at 0 V vs. RHE for the n + p-Si/Al 2 O 3 /AgP 2 photocathode (Supplementary Fig. 38 ). With the addition of AgP 2 cocatalyst, the lifetime of the decay ( t 1/2 ) is increased from 8.7 to 64.5 µs due to capture of the electrons by AgP 2 . In summary, AgP 2 NCs show a remarkable 0.3 V decrease in overpotential for CO generation compared to the benchmark Ag catalyst. The AgP 2 NCs achieve a maximum Faradaic efficiency of 82% for CO production and a wide CO:H 2 ratio from 1:3 to 5:1 within an overpotential window of 500 mV. DFT calculations reveal a threefold energy barrier decrease for the formate intermediate formation step compared to Ag, resulting in a high CO:H 2 ratio at low overpotential. A n + p-Si/Al 2 O 3 /AgP 2 photocathode exhibits an impressive onset potential of 0.2 V vs. RHE for PEC CO 2 -to-CO reduction and a maximum FE CO of 67% at −0.2 V vs. RHE. Chemicals and materials Silver acetate (97%), oleylamine (OAm, tech. 70%), oleic acid (OA, tech. 90%), 1-octadecene (ODE, tech. 90%), and Nafion 117 solution were purchased from Sigma-Aldrich. Tris(trimethylsilyl)phosphine ((Me 3 Si) 3 P, 98%) dissolved in hexane (10 wt%) was purchased from Stream Chemicals. Commercial carbon black was obtained from FuelCellStore. Si wafers with a resistivity of 1–100 Ω cm (p-type, B-doped, (100) orientation, prime grade, 500 μm thickness, 100 mm diameter) were obtained from University Wafer. Synthesis of sub-4 nm silver phosphide (AgP 2 ) NCs Silver acetate (0.5 mmol, 0.0835 g), OAm (6 mL), OA (1 mL), and ODE (6 mL) were added into a 50-mL three-neck, round bottom flask containing a stirring bar. This solution was placed under vacuum at 60 and 120 °C to degas for 30 min, respectively, to remove the low boiling point impurities and oxygen. The solution was placed under nitrogen and heated to 180 °C. Meanwhile, a second precursor solution comprising 2 mL (Me 3 Si) 3 P (10 wt% in hexane) and 1 mL ODE was degassed under vacuum and room temperature for 10 min in a 10 mL vial with a septum cap to remove hexane. The (Me 3 Si) 3 P solution was rapidly injected into the reaction flask at 180 °C and kept for 10 min at this temperature. Finally, the solution was maintained at 80 °C for 1 h to complete the Ostwald ripening and then cooled to room temperature. The reaction mixture was centrifuged at 3300 × g for 6 min The isolated precipitate was re-suspended in hexane, then acetone and methanol were added to create a 1:6:1 (v:v:v) hexanes:acetone:methanol solution to cause aggregation of the NCs. The resulting cloudy solution was centrifuged. This isolated solid was redissolved in hexane and the process repeated for an additional three times. Finally, the product was dispersed in hexane (2 mg/mL). For comparison, 10 nm AgP 2 NCs were synthesized similarly but the reaction time at 180 °C was 25 min instead of 10 min, 4 and 10 nm Ag NCs were synthesized by co-heating the precursors of silver acetate (0.5 mmol), 8 mL OAm, 0.5 mL OA at 180 °C for 20 min and 2 h, respectively. Materials characterizations Elemental analysis was performed using inductively coupled plasma mass spectroscopy (ICP-MS; Teledyne Leeman Labs). XRD patterns were obtained on an X-ray diffractometer (Bruker D2 Phaser) using Cu K α radiation. HRTEM was carried out on a Tecnai G2 F20 microscope at 200 or 300 kV. STEM and EDS were performed on a JEOL JEM 2200FS STEM/TEM microscope at an acceleration voltage of 200 kV equipped with a CEOS probe corrector (Heidelberg, Germany) to provide a nominal resolution of ~0.07 nm. A Bruker-AXS silicon drift detector (SDD) was used for all EDS elemental analysis. All colloidal samples for TEM measurements were prepared by ultrasonic dispersion in hexane and were dropcast onto copper grids covered with a carbon film. For the hybrid photocathode, the corresponding cross-sectional TEM sample was prepared by mechanical sectioning and polishing to a thickness of 20 µm. The polished film was further thinned until perforation by focused ion beam and measured by HRTEM (Tecnai G2 F20 microscope at 300 kV). XPS (Kratos Axis Ultra DLD, UK) was used to detect the chemical composition of the as-prepared samples. The binding energy was calibrated based on the C 1 s peak at 284.8 eV. Ultraviolet photoelectron spectroscopy (UPS) was performed using the same XPS instrument with a 165 mm hemispherical sector analyser. UPS was measured with a He I (21.2 eV) radiation source and a total energy resolution of 200 meV. Ag K-edge X-ray absorption fine structure (XAFS) measurements were made at the beamline 14W1 in Shanghai Synchrotron Radiation Facility (SSRF), China. The storage ring of SSRF was operated at 3.5 GeV with a current of 300 mA. The extended XAFS (EXAFS) data were processed according to the standard procedures using the WinXAS3.1 program. Theoretical amplitudes and phase-shift functions were calculated with the FEFF8.2 code using the crystal structural parameters of the Ag foil, Ag 2 O, and AgO. The parameters describing the electronic properties (e.g., correction to the photoelectron energy origin, E 0 ) and local structure environment including CN, bond distance ( R ), and Debye Waller (DW) factor around the absorbing atoms were allowed to vary during the fit process. The fitted ranges for k and R spaces were selected to be k = 3.0–11.5 Å −1 and R = 1–3 Å ( k 3 weighted), respectively. XANES calculation was based on self-consistent multiple-scattering (MS) methods, and was carried out using the FEFF8.2 code. The experimental absorption coefficients as a function of energies μ ( E ) were processed by background subtraction and normalization procedures, and reported as normalized absorption. Optical transmission measurements were performed using a Shimadzu 3600 UV–Vis–NIR spectrophotometer. To perform the optical absorption measurements, the sample was placed inside an integrating sphere and illuminated with white light from a 300 W xenon lamp. All light that was not absorbed was collected and measured using an Ocean Optics Jaz EL 200-XR1 spectrometer. Reflection data were calculated assuming that the absorbed, transmitted, and reflected light fractions sum to one. The femtosecond TA spectroscopy was carried out using PHAROS laser operating at 10 kHz coupled to an ORPHEUS optical parametric amplifier in tandem with a LYRA harmonic generator to produce the desirable wavelength for sample excitation. Relatively low pump intensity of 50 µW and 400 µJ cm −2 was used for femtosecond and microsecond TA experiment. A portion of laser output was split off to pump a sapphire crystal to generate a white light continuum for the probe beam in the region of 500–900 nm. Diffuse reflectance mode was adopted due to the non-transparent silicon photocathodes. The TA intensity is displayed as % absorption = (1− R / R 0 ) × 100, where R and R 0 are the probe pulse intensities with and without excitation, respectively. Catalyst inks preparation For the electrochemical measurements, the as-synthesized NC solution (5 mL at 2 mg/mL) was mixed with an equal amount by weight of Ketjen carbon (C) support (10 mg) in a 20 mL vial. This colloidal mixture was sonicated for 1 h to ensure complete distribution of NCs onto the carbon support. After evaporation of the volatile hexane, 5 mL of acetic acid was added to the NC/C solid and stirred for 12 h at 60 °C. The dispersion was cooled down to room temperature. Ethanol (8 mL) was added and the mixture was centrifuged at 3300 × g for 6 min This procedure was repeated three times. Finally, the solid NCs/C was then re-dispersed in a mixture of deionized water, isopropanol, and Nafion 117 solution (v:v:v = 4:2:0.05) to form a catalyst ink (2 mg/mL), 50 μL of which was deposited on the glassy carbon working electrode ( D = 5 mm) to form a catalyst film with a loading amount of about 0.5 mg/cm 2 and dried at ambient conditions. Pure Ketject carbon and AgP 2 /Ketject carbon mixtures with different ratios were also prepared using the same procedures for comparison. For the spin coating of the NC cocatalyst on the semiconductor, the concentration of ink solution was diluted to 0.5 mg/mL. Electrochemical measurements CO 2 electroreduction was carried out in a customized H-type cell separated by a Nafion 117 membrane with 0.5 M KHCO 3 . Each compartment contained 20 mL electrolyte and 10 mL headspace. A conventional three-electrode system, namely a disk shaped glassy carbon electrode (0.20 cm 2 ) coated with a catalyst was used as the working electrode, Ag/AgCl as the reference electrode, and graphite rod as the counter electrode, was employed for CO 2 reduction with a Reference 600 potentiostat (Gamry Instrument Inc.). The electrolyte solution was purged with high purity CO 2 gas for at least 1 h until a pH of 6.8 was reached before the electrochemical measurements. Before CO 2 electrolysis, the headspace was also purged for 20 min. The polarization curves were obtained with a scanning rate of 5 mV/s. Chronoamperometry was performed at a fixed potential for 2 h by maintaining a constant CO 2 flow rate. Gas-phase products were sampled every 30 min using a 50 µL gas-tight syringe (Hamilton). A gas chromatograph (GC, Agilent 6890) with a thermal conductivity detector was used for quantification. Liquid products were detected and quantified using a Bruker Avance 400 MHz NMR spectrometer. Typically, a 500 µL electrolyte was sampled after electrolysis and mixed with 100 µL D 2 O and 1.67 ppm DMSO. The electrode stability was tested by chronoamperometry under a constant potential of −0.8 V vs. RHE for 12 h. Electrochemical impedance spectroscopy under dark conditions was performed on a Reference 600 (Gamry Instrument Inc.) with the working electrode biased at a constant potential of −0.1 V vs. RHE, while sweeping the frequency from 10 5 to 0.1 Hz with a 10 mV AC dither. The EASA values of the as-prepared electrodes were evaluated by CV using the ferri-/ferrocyanide redox couple ([Fe(CN) 6 ] 3−/4− ) as a probe. Cyclic voltammetry was carried out in a nitrogen-purged 5 mM K 3 Fe(CN) 6 /0.1 M KCl solution with platinum foil as the counter electrode. EASA values were calculated using the Randles-Sevcik equation (Eq. (1)), 
    I_p = ( 2.36 × 10^5)n^3/2A D^1/2C υ ^1/2,
 (1) where I p is peak current (A), n = 1, D = 4.34 × 10 –6 cm 2 s −1 , A is the EASA (cm 2 ), C is the concentration of potassium ferricyanide (5 × 10 –6 mol cm −2 ), and υ is the scan rate (5 mV s −1 ). All potentials reported in this paper were converted from vs. Ag/AgCl to vs. RHE by adding a value of 0.197 + 0.059 × pH. Fabrication of hybrid photocathode Degenerately boron-doped Si wafers with a resistivity of 0.002 Ω cm −1 (p-type, 500 µm) were cut into 2 × 1.5 cm 2 pieces. The p-Si wafers were cleaned and etched in hydrofluoric acid to remove the native oxide and trace contaminants. The surface n-type doping of the p-Si wafers was treated with phosphorus from POCl 3 gas for 10 min at 900 °C [55] . We also prepared the control samples with different doping time (20 and 30 min). The backside of each p-Si-based photocathode was scratched and painted with a gallium indium eutectic for good electrical contact. The Al 2 O 3 surface protective layers were deposited on the n + p-Si by a GEMSTAR-6 ALD system. Trimethylaluminum (TMA) and distilled water (H 2 O) were used as precursors of Al and O, respectively. The ALD of Al 2 O 3 was carried out at a substrate temperature of 175 °C. Each precursor was held in the chamber for 2.2 s, followed by a 28 s nitrogen purge. The growth rate per cycle (GPC) was identified by X-ray reflectivity on films deposited on optically polished silicon wafers with a native surface oxide. The GPC was 1.2 Å for Al 2 O 3 . Next, the AgP 2 NC cocatalyst layer was deposited by layer-by-layer spin coating using 200 μL of the AgP 2 NCs solution (0.2 mg/mL) for each cycle. The spin coating was carried out at 1467 × g for 45 s. The optimized spin cycle for AgP 2 deposition is identified as one cycle. Different catalyst coverage was monitored by controlling the spin cycles of diluted AgP 2 ink. Finally, the hybrid photocathode was treated by annealing at 200 °C for 60 min in a tube furnace under a flow of N 2 . PEC measurements The photoelectrochemical activity of the photocathodes was measured in a home-made PEC reactor [56] with a three-electrode system using a Reference 600 potentiostat (Gamry Instrument Inc.). The prepared n + p-Si/Al 2 O 3 /AgP 2 served as the working electrode, a graphite rod as the counter electrode, and Ag/AgCl as the reference electrode. A Nafion 117 membrane was inserted into the PEC reactor to separate the working and counter electrodes. The electrolyte was a CO 2 -saturated 0.5 M KHCO 3 solution. A 300 W Xenon arc lamp (Newport) equipped with an AM-1.5G filter was used to simulate the solar spectrum. The light intensity was calibrated to 100 mW/cm 2 through a Newport 843-R power meter. The geometric area of the photocathode under light illumination was measured and maintained at nearly 1 cm 2 . The incident photoelectron conversion efficiency was measured by a specially designed IPCE system (Zolix Solar Cell Scan 100) with a 150 W Xe lamp and a monochromator (Oriel Cornerstone 130). For the interfacial charge transport characterization, CVs were recorded under dark or light illumination in a ferri/ferrocyanide solution which was made of 10 mM of both K 3 Fe(CN) 6 and K 4 Fe(CN) 6 in 1 M aqueous KCl.